Geometrically locked vortex lattices in semiconductor quantum fluids Macroscopic quantum states can be easily created and manipulated within semiconductor microcavity chips using exciton-photon quasiparticles called polaritons. Besides being a new platform for technology, polaritons have proven to be ideal systems to study out-of-equilibrium condensates. Here we harness the photonic component of such a semiconductor quantum fluid to measure its coherent wavefunction on macroscopic scales. Polaritons originating from separated and independent incoherently pumped spots are shown to phase-lock only in high-quality microcavities, producing up to 100 vortices and antivortices that extend over tens of microns across the sample and remain locked for many minutes. The resultant regular vortex lattices are highly sensitive to the optically imposed geometry, with modulational instabilities present only in square and not triangular lattices. Such systems describe the optical equivalents to one- and two-dimensional spin systems with (anti)-ferromagnetic interactions controlled by their symmetry, which can be reconfigured on the fly, paving the way to widespread applications in the control of quantum fluidic circuits. In systems described by the laws of quantum mechanics, continuity of the wavefunction implies that circulating flows assume quantized values called vortices. Vortex lattices were first predicted [1] and later observed [2] in type-II superconductors, in response to an externally applied magnetic field. In neutral quantum fluids, external rotation was used to generate vortex lattices in superfluids of helium [3] and later in atomic Bose–Einstein condensates (BECs) [4] . Recent proposals include the generation of honeycomb vortex-antivortex lattices through linear interference of three expanding BECs [5] . Such lattices have never been observed experimentally, although related techniques have been used to nucleate vortices in BECs [6] or vortex solitons in non-linear media that have been used as waveguides [7] and photonic crystals [8] . Recently a new type of macroscopic coherent state was observed in semiconductor microcavities [9] , where excitons in a quantum well strongly couple with photons confined between two mirrors producing quasiparticles called polaritons [10] . Polariton condensates have a finite lifetime and need to be constantly pumped, prompting extensive studies of the rich phenomena in out-of-equilibrium condensates [9] . This also makes it simple to shape the condensate flow [11] , [12] , [13] and sculpt the confinement potential [12] , [13] , [14] using the pump fields. Vortices were first observed in polariton condensates in highly inhomogeneous samples as a result of pump and decay processes which pin them to defects [15] , [16] . Recently it has also proved possible to generate vortices by coherent resonant injection [17] , [18] together with flow against defects [19] , [20] . However, no observation of the predicted [21] spontaneous regular distribution of vortices in a lattice has yet been reported. Being neutral systems, polariton condensates cannot produce vortex lattices in response to a magnetic field, but theoretical proposals suggest generating such lattices using harmonic traps [15] or resonant laser injection [22] , [23] . Here we show that it is possible to generate a stable lattice of vortices, containing vortex sub-lattices of opposite winding numbers, by appropriately engineering the condensate wavefunction through shaping the pumping configuration. These are sustained inside next-generation high-quality samples, where the extremely low disorder permits polaritons to propagate laterally without being scattered, and allows them to respond to imposed rotational and translational symmetries which phase-lock different condensates through a new geometrical process. The vortices observed are stable for many minutes, independent of precise position on the microcavity, and the continuously replenished lattices are directly seen in continuous-wave experiments. A different regime observed at higher polariton densities reveals the non-linear dynamics of topological defects that move inside guides defined by the geometry. Honeycomb stable vortex lattice First, we incoherently and continuously pump the microcavity sample with three 1 μm diameter laser beams equidistant from each other. Each pump spot generates an electron-hole plasma that rapidly cools and scatters into polaritonic modes, whose Coulomb repulsion locally blueshifts their energies by Δ at each pump spot position. The slow escape from the cavity of their photonic components allows the polariton wavefunctions to be measured. With equal powers in each pump, above a threshold (typically 5 mW per spot) a phase transition occurs, where the polariton energy distribution suddenly collapses from thermal to a single mode, followed by a non-linear increase of the emission intensity ( Supplementary Fig. S1 ). Under suitable pumping conditions ( Supplementary Fig. S2 ), interference patterns appear in the region where the condensates overlap between the three pump spots ( Fig. 1a ), with a characteristic honeycomb structure. Such a honeycomb density pattern is predicted to support a stable vortex lattice [21] . To confirm this, we extract the condensate phase using Fourier transform filtering applied to interference images ( Fig. 1c ) generated in a Mach–Zehnder interferometer (see Methods ). The resultant phase image ( Fig. 1b ) shows up to 50 vortices and antivortices located at the vertices of the honeycomb. Each vortex is surrounded by three vortices of opposite winding number, and so the hexagonal lattice can be seen as two Abrikosov-like triangular lattices [1] of opposite sign ( Fig. 1e ). The lattice is highly coherent over tens of microns ( Fig. 1d ) with interference visibilities over 50%, whereas the non-emissive vortex cores are seen as points of zero coherence with undefined phase. 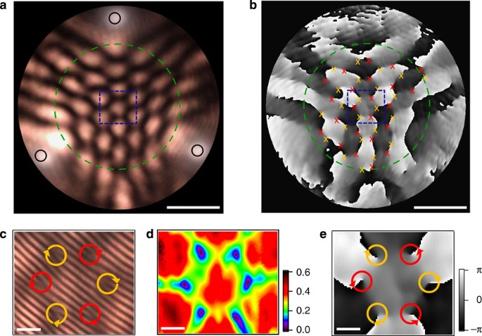Figure 1: Honeycomb vortex-antivortex lattice. (a) Intensity and (b) phase image of the polariton emission showing the honeycomb density pattern between the three excitation spots (black circles) with vortices (red crosses) and antivortices (orange crosses) marked. Scale bars, 5 μm. (c) Interference image of the region inside the dashed blue rectangle ina, showing vortices (red anticlockwise circles) and antivortices (orange clockwise circles) at the vertices of the triangular sub-lattices. (d) First-order coherence function,g(1), extracted fromc. (e) Expanded phase map of the dashed blue rectangle inbagain showing vortices and antivortices. Each spot is pumped with 14 mW for all the images. Scale bars, 1 μm (inc–e). Figure 1: Honeycomb vortex-antivortex lattice. ( a ) Intensity and ( b ) phase image of the polariton emission showing the honeycomb density pattern between the three excitation spots (black circles) with vortices (red crosses) and antivortices (orange crosses) marked. Scale bars, 5 μm. ( c ) Interference image of the region inside the dashed blue rectangle in a , showing vortices (red anticlockwise circles) and antivortices (orange clockwise circles) at the vertices of the triangular sub-lattices. ( d ) First-order coherence function, g (1) , extracted from c . ( e ) Expanded phase map of the dashed blue rectangle in b again showing vortices and antivortices. Each spot is pumped with 14 mW for all the images. Scale bars, 1 μm (in c – e ). Full size image This specific pattern is described by a single wavefunction coherent over tens of microns. It is an intricate superposition of wavevectors flowing out from each pump spot and slowing down at the neighbouring ones, with magnitude at each point given by the condensate energy, E c , and the local blueshift, Δ( r ) (see Supplementary Discussion and Fig. 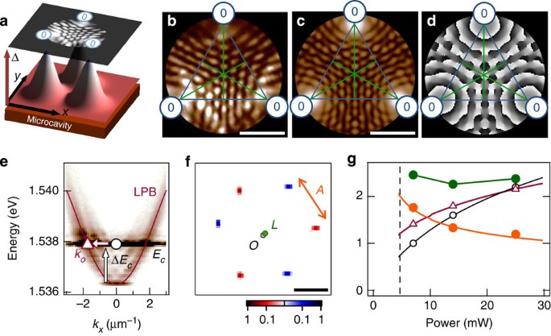Figure 2: Lattice control and geometric locking. (a) Schematic landscape of the blueshift-induced potential Δ(r) underlying the geometrically phase-locked vortex lattice. (b) Measured polariton emission for 25 mW excitation power per spot, with green lines crossing at the spots centroid. Simulated wavefunction (c) density and (d) phase, showing vortices and the equal phases at each pump spot position (represented by blue zeros inside circles). Scale bars, 10 μm. (e) Energy dispersion of the region inside the dashed green circle inFig. 1a, showing the fitted LPB (purple line). Blueshift of the condensate energy (ΔEc, black circles) is set by the blueshift at the excitation spots, with condensate momentum at the spots centroid (ko, purple triangles) given byk(r)=K[ΔEc] (equation 1). (f) Normalized circulation calculated fromFig. 1e, showing the separation (A) between adjacent vortices, with lattice centroid (L) and spots centroid (O). Scale bar, 1 μm. (g) Power dependence of the lattice energy (ΔEc, in meV, black circles) with logarithmic fit (black line), measured lattice maximum momentum (ko, in μm−1, purple triangles) with prediction based on the dispersion (purple line), measured lattice separation (A, μm, orange circles) with prediction (orange line) from, and ferro offset (F=|L−O|/[2π/k0], in %, green circles). Dashed line at condensation threshold. 2a ), Figure 2: Lattice control and geometric locking. ( a ) Schematic landscape of the blueshift-induced potential Δ( r ) underlying the geometrically phase-locked vortex lattice. ( b ) Measured polariton emission for 25 mW excitation power per spot, with green lines crossing at the spots centroid. Simulated wavefunction ( c ) density and ( d ) phase, showing vortices and the equal phases at each pump spot position (represented by blue zeros inside circles). Scale bars, 10 μm. ( e ) Energy dispersion of the region inside the dashed green circle in Fig. 1a , showing the fitted LPB (purple line). Blueshift of the condensate energy (Δ E c , black circles) is set by the blueshift at the excitation spots, with condensate momentum at the spots centroid ( k o , purple triangles) given by k ( r )= K [Δ E c ] (equation 1). ( f ) Normalized circulation calculated from Fig. 1e , showing the separation ( A ) between adjacent vortices, with lattice centroid ( L ) and spots centroid ( O ). Scale bar, 1 μm. ( g ) Power dependence of the lattice energy (Δ E c , in meV, black circles) with logarithmic fit (black line), measured lattice maximum momentum ( k o , in μm −1 , purple triangles) with prediction based on the dispersion (purple line), measured lattice separation ( A , μm, orange circles) with prediction (orange line) from , and ferro offset ( F =| L − O |/[2 π / k 0 ], in %, green circles). Dashed line at condensation threshold. Full size image where K [ E ] is the inverse dispersion relation ( Fig. 2e ) and Δ E c = E c − E LPB , the condensate energy with respect to the bottom of the unperturbed lower polariton branch (LPB). Polaritons are created with k =0 at each pump spot and accelerate outwards through decreasing blueshifts at larger distances [12] , [13] , with Δ( r >10 μm)=0. In the centre between the three pumped spots (spots centroid, O ) the wavefunction is thus the superposition of three k o vectors at 120° to each other, directed out from each pump spot ( Supplementary Fig. S3 and Supplementary Discussion ), whose linear combination generates the honeycomb lattice [5] . However, the separation between adjacent vortices is not constant over the lattice as the magnitude and direction of each of the three k vectors changes spatially according to equation (1). For instance, as the blueshift at each pump spot increases with pump power, the condensate energy increases, increasing k o , and thus decreasing the spacing between central vortices, A . ( Fig. 2f ). The non-linear condensate properties can thus be used to stretch the vortex lattice spacing, here by over 50% from 1.2 to 1.8 μm. Ferromagnetic coupling To fully describe the lattice wavefunction, simulations are performed using a simple form of the mean field model of polariton condensates [6] , [15] through the complex Ginzburg–Landau equation, which includes both dissipation and pumping, where U 0 is the strength of polariton interactions, κ is their decay, and the details of pumping are included in . Here, the dimensionless parameter η describes the energy relaxation via interactions of condensate and reservoir, γ is the gain and Γ is a nonlinear coefficient describing the non-linear reduction of pumping efficiency at large polariton densities. Parameters are the same as in [21] (with a single component only), and the radius of the pumping spots is 1 μm. Numerical solution of this equation for three equally spaced pump spots reproduces the vortex lattice found in experiments ( Fig. 2c ). It gives a wavefunction with the same phase at each pump spot position ( Fig. 2d ), independent of the initial state, and hence the central bright lobe appears at O , the spots' centroid ( Fig. 2c ). This is the only solution that is invariant under interchange of the spot positions, and so is geometrically imposed by the pumping configuration. However, it is spontaneously chosen by the condensate system because the phase carried by the pumping laser is completely lost during the relaxation processes. The pumped spots acquire the same spontaneous phase (or equivalently, pseudo-spin) and our triangular configuration avoids pseudo-spin frustration by insisting on ferromagnetic nearest neighbour interactions. Thus, the vortex lattice is controlled by the pseudo-spin symmetry of the optically induced condensates, analogous to ferromagnetism in two-dimensional (2D) spin systems. The precise vortex positions are extracted by calculating the circulation, from the phase map, where is the measured local fluid velocity. For any contour around a vortex the quantum of circulation is Γ =± h / m . Using Stokes theorem, we thus generate a normalized circulation for each pixel of area d S ( Fig.2f ) given by , where the local vorticity, ω = × v . The separation (as a fraction of the periodicity 2 π / k o ) between the centroids of this vortex lattice ( L ) and the pumped spots ( O ) quantifies the deviation from perfect ferromagnetic coupling (that is, the state where the phase at each pump spot is identical). For three different powers, this ‘F offset’ is found to be always below 3% ( Fig. 2g ) for periods of time of many minutes much longer than , showing that ferromagnetic coupling is always dominant in the triangular geometry. The stability of the lattice persists then due to the non-linear geometric phase locking of the free condensate phase of each pumped spot. This implies that rich spin phenomena such as ladder magnets [24] may be directly investigated in the polariton system. Square bistable lattices Lattices with different geometry can be simply engineered by changing the number and position of pump spots. Square lattices are created when pumping the sample with four spots placed at the vertices of a square ( Fig. 3 ). However, unlike the three-spot geometry in which the condensates lock with the same phase, numerical solutions of equation (2) show two different possible relative phases between nearest neighbour condensates depending on initial conditions: either 0 ( Fig. 3a ) or π ( Fig. 3c ). These are analogous to ferromagnetism (F) and anti-ferromagnetism (AF), respectively, in 2D spin systems ( Fig. 3h ), and can again be distinguished in experiments by looking at the polariton density at the centroid between the spots: as seen in experiments, F-coupled condensates have an antinode at the centre ( Fig. 3e ) whereas AF-coupled have a node ( Fig. 3g ). This bistable pseudo-spin configuration, which can then correspond to a qubit or an interferometer, can potentially be manipulated through direct laser excitation, as well as in lithographically patterned samples [25] . 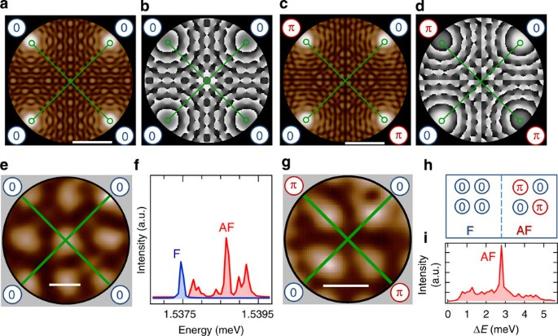Figure 3: Square lattice and pseudo-spin symmetry. (a–d) Numerical solutions of equation (2) under different initial noise, giving F (a,b) or AF (c,d) lattices. Scale bars, 10 μm. (e,g) Observed polariton density at main energy peak, 1.5374, eV and 1.5386, eV, respectively, for 12 mW and 40 mW excitation power per spot, respectively, with the intersection between the two green lines marking the spots centroid. Scale bars, 2 μm. (f) Lattice spectra for two different powers, 12 mW (blue line) and 40 mW (red line), with main peaks classified according to the polariton density at the spots centroid. (h) Schematic ferromagnetic (F) and antiferromagnetic (AF) stable pseudo-spin configurations (numbers inside circles represent the condensate phase at each pump spot). (i) Spectra of simulated square lattice. Figure 3: Square lattice and pseudo-spin symmetry. ( a – d ) Numerical solutions of equation (2) under different initial noise, giving F ( a , b ) or AF ( c , d ) lattices. Scale bars, 10 μm. ( e , g ) Observed polariton density at main energy peak, 1.5374, eV and 1.5386, eV, respectively, for 12 mW and 40 mW excitation power per spot, respectively, with the intersection between the two green lines marking the spots centroid. Scale bars, 2 μm. ( f ) Lattice spectra for two different powers, 12 mW (blue line) and 40 mW (red line), with main peaks classified according to the polariton density at the spots centroid. ( h ) Schematic ferromagnetic (F) and antiferromagnetic (AF) stable pseudo-spin configurations (numbers inside circles represent the condensate phase at each pump spot). ( i ) Spectra of simulated square lattice. Full size image We find effects unique to polariton liquids. If non-linear effects are not taken into account, stationary lattices form and no vortices are expected to appear at the spots centroid ( Fig. 3b and Supplementary Fig. S4a,b ). In this case each intensity lobe would have a constant phase with abrupt π shifts localized in the zero density regions. However, under high excitation powers, an AF-coupled lattice is accompanied with weaker energy sidebands ( Fig. 3f ) that indicate non-linear temporal dynamics. This is confirmed by extracting the spatio-temporal behaviour from experiments (see Supplementary Discussion ), which shows that dark soliton instabilities generate vortex-antivortex pairs. Although the precise trajectory of each topological defect is stochastic, these vortices are completely constrained to the square grid defined by density minima. Such instabilities are observed in both experiments and simulations ( Supplementary Figs S5–S7 ). Modulational instabilities that nucleate vortex pairs also resemble effects in non-linear optical media [26] . This pump geometry thus provides a way to generate periodic 2D structures in polariton condensates, with no need of a built-in periodic potential [27] . The interacting topological defects move around on the dark lines in this square matrix, while quantized values of vortex charge can also be restricted to specific positions in this lattice (see Supplementary Fig. S4c–f ). Controlling further such vortices will pave the way towards manipulation of quantum fluidic circuits [25] . The vortex lattices presented here are created with no need of global stirring or external rotation, and the vortex/antivortex pairs yield no global angular momentum. They are thus markedly distinct from lattices due to global phase symmetries described in [4] and present a close analogy to the formation of vortex solitons in Kerr non-linear self-defocusing media [7] . The phase locking between separately pumped condensates is a key ingredient for the lattice generation and stability, but here the locking mechanism has no relation with previously reported Josephson tunnelling in disorder-induced trapped condensates [28] , [29] . Instead, each of the pumped spots is resonantly pumped by the outflow from the neighbouring condensates inducing mode-locking to the same energy. As the phase of the polariton fluids has no relation to that of our pumping lasers, the lattice is a purely non-linear polaritonic effect spontaneously emerging from the optically induced potential. Sample The sample, held at 10 K in a cold finger cryostat, consists of a 5 λ /2 Al 0.3 Ga 0.7 As distributed Bragg reflector microcavity with 32 (35) pairs of Al 0.15 Ga 0.85 As/AlAs layers of 57.2 nm/65.4 nm in the top (bottom) mirrors. It has four sets of quantum well regions, each containing three 10 nm thick GaAs quantum wells separated by 10 nm thick Al 0.3 Ga 0.7 As layers, placed at the antinodes of the cavity electric field. The high cavity quality factor ( Q >16,000 measured, and simulated photon lifetime of 9 ps) yields a characteristic Rabi splitting of 9 meV. We choose the detuning between photonic and excitonic modes to be −3 meV by scanning the cavity wedge. Experiment setup A Ti:sapphire single-mode continuous-wave laser pumps the sample at 750 nm (at the first spectral dip above the stop band) with 1 μm diameter spots through a 0.7 numerical aperture lens, which also collects light emitted by the sample. Magnified real-space and momentum-space images are recorded on a Si CCD or analysed spectrally with a 0.55-m monochromator and liquid nitrogen-cooled CCD. Interferometry To generate a reference wave for interferometry that is sensitive only to the relative condensate phases (as their absolute phase is freely diffusing), we use condensate emission from 40 μm outside the lattice, behind one of the pump spots. In this technique, introduced in [17] , [18] , a small portion of this constant phase reference wave is magnified, and interfered with the sample emission in a Mach–Zehnder interferometer (giving for instance Fig. 1c ). As a control, this reference wave is confirmed to give parallel fringes with no artefacts when interfering it with corresponding regions behind the other pumped spots. Phase and coherence images are then obtained when taking the first-order diffraction components from the Fourier-transformed interference images. The argument of the back-transformed inverse Fourier transforms gives an image of the condensate phase, whereas the intensity image gives the fringe visibility and hence the first-order coherence. The latter is normalized to the product of the intensity from each interferometer arm. How to cite this article: Tosi, G. et al . Geometrically locked vortex lattices in semiconductor quantum fluids. Nat. Commun. 3:1243 doi: 10.1038/ncomms2255 (2012).